Single-crystal field-effect transistors of new Cl2-NDI polymorph processed by sublimation in air Physical properties of active materials built up from small molecules are dictated by their molecular packing in the solid state. Here we demonstrate for the first time the growth of n-channel single-crystal field-effect transistors and organic thin-film transistors by sublimation of 2,6-dichloro-naphthalene diimide in air. Under these conditions, a new polymorph with two-dimensional brick-wall packing mode ( β -phase) is obtained that is distinguished from the previously reported herringbone packing motif obtained from solution ( α -phase). We are able to fabricate single-crystal field-effect transistors with electron mobilities in air of up to 8.6 cm 2 V −1 s −1 ( α -phase) and up to 3.5 cm 2 V −1 s −1 ( β -phase) on n -octadecyltriethoxysilane-modified substrates. On silicon dioxide, thin-film devices based on β -phase can be manufactured in air giving rise to electron mobilities of 0.37 cm 2 V −1 s −1 . The simple crystal and thin-film growth procedures by sublimation under ambient conditions avoid elaborate substrate modifications and costly vacuum equipment-based fabrication steps. New organic semiconductor molecules as well as device fabrication technologies afforded an impressive development in the field of organic field-effect transistors [1] , [2] , [3] . As the morphology of organic semiconducting thin films on a dielectric layer has a crucial impact on the charge transport properties and determines the device performance, for the demand of high device performance, many studies have been devoted to manufacture highly ordered crystalline films, which has been effectively solved by interface engineering and the improvement of fabrication processes, for examples, by introduction of self-assembled monolayers, annealing and inkjet printing technology [4] , [5] , [6] , [7] , [8] . However, despite the well-known fact that polymorphism in thin films is not easy to avoid and different phases have a great impact on the charge carrier transport properties, only for few organic semiconductors, detailed studies on crystalline polymorphs investigated in organic thin-film transistors (OTFTs) are available [9] , [10] , [11] , [12] , [13] , [14] , [15] . The reason might be that individual pure single crystalline phases are difficult to prepare in thin films and challenging analytics are needed to distinguish coexisting polymorphs in various domain structures, not to mention the impact of grain boundaries between domains of different phases on the charge carrier transport. In contrast to thin films, single crystals with perfect molecular order are free of grain boundaries on relevant length scales and ideally suited for the investigation of the intrinsic properties of organic semiconductors to correlate charge transport with respect to molecular arrangement [16] , [17] . In addition, phase transitions between different polymorphs can be followed by single-crystal X-ray structure analysis [18] , [19] , [20] , [21] . Because of the experimental challenges of such studies, however, knowledge on such phase transition and their impact on electrical transport properties has only been acquired for few organic materials [22] , [23] , [24] , [25] , [26] , [27] , [28] , [29] . For examples, four polymorphs have been reported for pentacene single crystals [22] , [23] and four different phases and their crystal structures have been revealed for dibenzo-tetrathiafulvalene (DB-TTF) [24] , which, however, were so far not investigated with respect to their charge carrier mobility in single-crystal field-effect transistors (SCFETs). For tetrathiafulvalene (TTF) [25] , diindenoperylene [26] , [27] and dithiophene-tetrathiafulvalene (DT-TTF) [28] , phase transitions have also been reported, and charge transport properties were explained by the crystal structure of respective phases. However, a deeper insight into the process and mechanism of such structural phase transitions and their relation to charge carrier transport combined with temperature-dependent measurements has so far been elusive, despite of their great influence to devices’ mobility and stability. This holds in particular true for electron transport materials (n-channel organic semiconductors) whose sensitivity towards ambient gases and humidity is far more pronounced than for above-discussed hole transport materials pentacene, diindenoperylene, TTF, DB-TTF and DT-TTF. In recent years, our group as well as others reported a significant number of naphthalene diimide (NDI)-based thin film transistor studies demonstrating excellent and stable n-channel operation even in air that can be attributed to a large electron affinity and close π-stacking [30] , [31] , [32] , [33] , [34] , [35] , [36] . For NDI small molecules, the highest mobilities could be obtained for thin-film transistors of DI-DTYM2 (3.5 cm 2 V −1 s −1 ) [34] and for single-crystal transistors of Cl 2 -NDI (8.6 cm 2 V −1 s −1 ) [35] , respectively, under ambient operation. In this article, we report on SCFETs and OTFTs of N,N′ -bis-(heptafluorobutyl)-2,6-dichloro-1,4,5,8-naphthalene tetracarboxylic diimide (Cl 2 -NDI) that can even be manufactured by simple sublimation under ambient conditions. To the best of our knowledge, this is the first example of n-channel organic transistors grown by simple sublimation in air. In addition, we discover that the Cl 2 -NDI crystals obtained by sublimation constitute a so far not crystallographically characterized polymorph ( β -phase) whose electrical properties are distinct from the already reported α -phase obtained by crystallization from solution at room temperature. Combining XRD (X-ray diffraction), DSC (differential scanning calorimetry), POM (polarization optical microscopy) and ultraviolet–visible spectroscopy, we investigate the structural phase transition between the more dense herringbone and the less dense two-dimensional brick-wall phases and their temperature-dependent SCFET properties. Crystal growth and structure analysis of polymorphs Although our recently reported procedure towards high mobility SCFETs was based on ribbon-shaped crystals of Cl 2 -NDI grown by the drop-casting method on n -octadecyltriethoxysilane (OTES)-modified substrate and by solvent evaporation method ( Supplementary Fig. 1 ) [35] , the low molecular weight of Cl 2 -NDI ( M =699 g mol −1 ) and excellent air-stability suggested that this molecule might be processed by simple sublimation under ambient conditions. With the setup shown in Fig. 1a , ribbon-shaped crystals with tens of micrometre size could indeed be grown on various substrates like Si/SiO 2 by sublimation at ambient pressure in air. The thin single crystals with green colour were selected by optical microscopy and were further investigated by atomic force microscopy (AFM), showing smooth surfaces and a thickness of less than 20 nm ( Fig. 1b,c ). 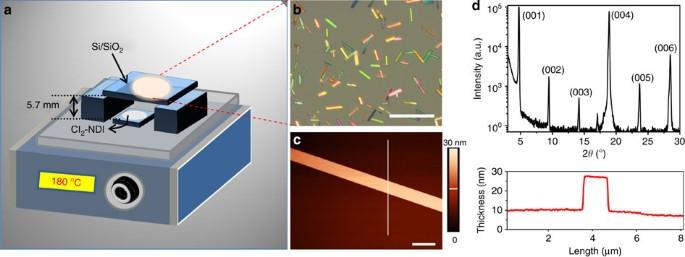Figure 1: Single crystal growth by simple sublimation in air. (a) Schematic drawing of the applied setup for crystal growth on Si/SiO2substrates. (b) Optical microscopy image of theβ-phase single crystals grown on Si/SiO2substrate. Scale bar, 200 μm. (c) AFM image and cross-section thickness analysis of a representative single crystal. Scale bar, 2 μm. (d) Corresponding XRD pattern of the crystals inb. Figure 1: Single crystal growth by simple sublimation in air. ( a ) Schematic drawing of the applied setup for crystal growth on Si/SiO 2 substrates. ( b ) Optical microscopy image of the β -phase single crystals grown on Si/SiO 2 substrate. Scale bar, 200 μm. ( c ) AFM image and cross-section thickness analysis of a representative single crystal. Scale bar, 2 μm. ( d ) Corresponding XRD pattern of the crystals in b . Full size image To our surprise, powder X-ray diffraction analysis in reflective geometry at 298 K of these crystals grown on Si/SiO 2 or OTES-modified Si/SiO 2 substrate by sublimation showed a completely different diffraction pattern ( Fig. 1d : diffraction peaks at 2 θ =4.74°, 9.47°, 14.1°, 18.9°, 23.7° and 28.5°, corresponding to a layer spacing of 18.64 Å) compared with the previously reported single crystals grown from solution on OTES-modified Si/SiO 2 substrate ( Supplementary Fig. 2 : diffraction peaks at 7.72°, 15.48° and 23.27°, corresponding to a layer spacing of 11.84 Å) [35] , thus yielding first evidence that a different crystallographic phase has been obtained by sublimation, as will be confirmed by the detailed comparison of their single-crystal structures below ( Supplementary Data 1–3 ). In the following, we will denote this polymorph by β -phase, whereas the formerly described phase [35] with smaller layer spacing is called α -phase. Based on these new results, we can now also re-assign the hitherto reported vacuum-processed thin-film transistors [31] to relate to the β -phase molecular packing arrangement. Crystals of sufficient size for single-crystal X-ray analysis of the new β -phase could be obtained by sublimation in a quartz tube at ambient pressure in air (for details, see Supplementary Fig. 3a ). These crystals appeared as thin slices with yellowish colour of millimetre size dimension ( Supplementary Fig. 3b ). Because the formerly published single-crystal data for the α -phase were of low quality [31] , we grew new crystals of this polymorph by the solution evaporation method ( Supplementary Table 1 and Supplementary Fig. 1b ). The colourless α -phase crystals belong to the monoclinic system, space group P2 1 / c , with two symmetrically equivalent molecules in the unit cell ( Supplementary Fig. 4 ). The torsion angle between fluoroalkyl chain and longitudinal direction of the NDI skeleton is 129.7° ( Fig. 2a ). The molecules arrange in a herringbone packing motif with the slipping angle of 62° along the c -axis. Nearly half of each NDI molecular skeleton overlaps with the adjacent molecule at a close π-stack distance of 3.27 Å in a slipped molecular arrangement in the crystal structure measured at 100 K ( Fig. 2b and Supplementary Fig. 5 ). The value of d 100 (11.84 Å) that was also found for the layer spacing is far less than the molecular size (~18 Å) because of the interdigitation and tilting of densely packed fluoroalkyl chains with F···F and F1···O1–C5 interactions ( Fig. 2c and Supplementary Fig. 2 ) [35] . 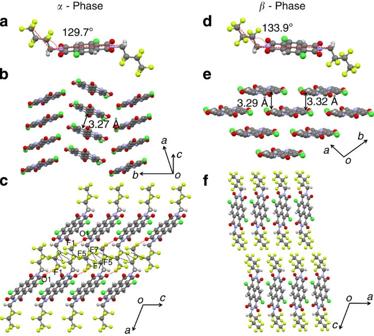Figure 2: Crystal structures of both polymorphs at 100 K. Molecular structure of Cl2-NDI in (a)α-phase and (d)β-phase. Crystal packing structures of (b) herringbone packing mode with π–π distance of 3.27 Å and the slipping angle of 62° forα-phase, and (e) two-dimensional brick-wall packing with π–π distances of 3.29 Å and 3.32 Å in the (ab)-plane, corresponding to slipping angles of 41° and 32° forβ-phase, respectively (for clarity, −CH2C3F7omitted). Crystal packing structures of (c)α-phase and (f)β-phase Cl2-NDI with tilt angles of about 67° and 90° on the substrate, respectively. The red, green, blue, grey, white and yellow coloured atoms represent O, Cl, N, C, H and F, respectively. Figure 2: Crystal structures of both polymorphs at 100 K. Molecular structure of Cl 2 -NDI in ( a ) α -phase and ( d ) β -phase. Crystal packing structures of ( b ) herringbone packing mode with π–π distance of 3.27 Å and the slipping angle of 62° for α -phase, and ( e ) two-dimensional brick-wall packing with π–π distances of 3.29 Å and 3.32 Å in the ( ab )-plane, corresponding to slipping angles of 41° and 32° for β -phase, respectively (for clarity, −CH 2 C 3 F 7 omitted). Crystal packing structures of ( c ) α -phase and ( f ) β -phase Cl 2 -NDI with tilt angles of about 67° and 90° on the substrate, respectively. The red, green, blue, grey, white and yellow coloured atoms represent O, Cl, N, C, H and F, respectively. Full size image The β -phase crystals, measured also at 100 K, belong to the triclinic system, space group P−1 with a =5.1862(4) Å, b =6.3422(5) Å, c =18.4245(15) Å and α =98.7225(18)°, β =91.6531(19)°, γ =109.6865(18)°. Just one molecule exists in the unit cell with a torsion angle of 133.9° between the fluoroalkyl chains and the longitudinal direction of the NDI skeleton ( Fig. 2d ). In contrast to the herringbone structure of α -phase, β -phase molecules exhibit a two-dimensional brick-wall packing arrangement. The π-stacking distances between aromatic scaffolds of two adjacent molecules are 3.29 and 3.32 Å, with slipping angles of 41° and 32°, respectively ( Fig. 2e and Supplementary Fig. 5 ). The unit cell distance along the c -axis of 18.73 Å is well in agreement with the molecules’ length (~18 Å), suggesting that β -phase Cl 2 -NDI molecules also adopt an edge-on conformation with the molecular long axis upright on the substrate as observed for the α -phase and supported by XRD data ( Fig. 1d ). In contrast to the more tilted arrangement for α -phase, β -phase molecules are standing upright along the [001] direction with an angle of almost 90° and there are almost no interactions between adjacent molecular layers along the direction of long molecular axis ([001] direction, Fig. 2f ). A more detailed comparison is presented in Supplementary Table 1 , regarding crystal data and structure refinement parameters for the two different polymorphs of Cl 2 -NDI. According to their respective crystal structure at 100 and 200 K (see Supplementary Table 1 ), the two phases feature pronounced differences in their anisotropic thermal expansion behaviour. The c -direction of the α -phase and the a -direction of the β -phase show similar thermal expansion coefficients of α c =1.4 × 10 −4 K −1 and α a =1.3 × 10 −4 K −1 , respectively, which are presumably related to the comparable interaction strength and distance between NDI-cores in both morphologies (see Fig. 2c,f ). In contrast, the expansion coefficient along the a -axis of the α -phase α a =0.1 × 10 −4 K −1 is about one order of magnitude smaller than the corresponding value along the c -direction of the β -phase α c =1.6 × 10 −4 K −1 . This observation becomes clear considering the interlocked heptafluorobutyl groups of adjacent molecules in the α -phase, which impose a severe constraint on the spatial expansion at elevated temperatures. As a result of the pronounced thermal expansion along the a - and c -axes of the β -phase in combination with a weak intermolecular interaction, the b -direction shows even a slight compression upon heating α b =−0.2 × 10 −4 K −1 , which refers to a superimposed rotation of molecules [37] . A comparable amplitude, however, different in sign is observed for the thermal expansion coefficient along the b -direction of the α -phase α b =0.5 × 10 −4 K −1 . Remarkably, extrapolating the temperature-dependent unit cell volume of the two phases under the assumption of linear thermal expansion and angular conservation yields to a similar volume of 582 Å 3 per molecule at a crossover temperature of about 241 K. This value might be considered as reference temperature for the intrinsic α - to β -phase transition without superimposed effects by latent heat or kinetic hindrances. Phase transition between α - and β -phase Although at any given temperature and pressure, only one polymorph corresponds to the minimum in free energy and can be regarded as the thermodynamically stable phase, it is very challenging to clarify the phase diagram because of the high activation barriers encountered in the structural transformation of molecular crystals [15] , [19] , [22] , [23] , [24] , [25] . On the other hand, besides temperature, the solvent also plays an explicit role in the crystal nucleation and growth dynamics in solution and therefore many crystals formed in solution correspond to metastable polymorphs [9] , [10] , [11] , [12] , [13] , [14] , [15] , [18] , [19] , [20] , [21] , [22] , [23] , [24] , [25] , [26] , [27] , [28] , [29] . For Cl 2 -NDI, regardless of the utilization of pure or mixed solvents (CHCl 3 , CH 2 Cl 2 , chlorobenzene, CH 3 OH, THF, hexane), the crystals grown from solution are always colourless ribbon-shaped crystals, whose packing arrangement was confirmed as α -phase by XRD ( Supplementary Fig. 2 ). Next, to study the effect of temperature, α -phase ribbon-shaped crystals of micrometers size were heated from 25 to 180 °C on a quartz substrate with a heating rate of 10 K min −1 . Under the POM, no obvious changes occurred when heating the sample up to 160 °C in air ( Fig. 3a and Supplementary Fig. 6a–f ) and the presence of a single crystallographic phase, namely the α -phase could be confirmed by powder XRD analysis ( Fig. 3b ). Accordingly, when the temperature is lower than 160 °C, just (h00) peaks could be observed ( Fig. 3b , black lines). However, when the temperature exceeded 160 °C small crystals appeared and grew larger to display a plate shape at 180 °C ( Fig. 3a and Supplementary Fig. 6g–i ). Analogous temperature-dependent wide-angle X-ray scattering experiments of the α -phase crystals showed the same behaviour but additionally peaks of different crystal planes could be observed (see Supplementary Fig. 7 ). Concomitant with these changes the intensity of the (h00) peaks for the α -phase gradually decreased and a new series of (00l) peaks corresponding to the β -phase started to appear whose intensity increased with increasing temperature. Between 160 and 170 °C crystals of both phases coexisted ( Fig. 3b , blue lines). Because α -phase crystals are ruptured and the new β -phase just starts to form, the intensity of peaks for both phases are only very weak (for clarity, the intensity of peaks is magnified by a factor of 10!). With further increase in temperature, the formation of the β -phase is completed and the (h00) peaks of the α -phase all disappear, accompanied by an increase in intensity of (00l) peaks of β -phase ( Fig. 3b , red lines). 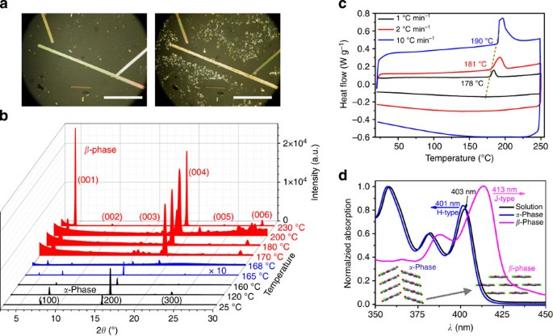Figure 3: Observations upon phase transformation fromα-phase toβ-phase. (a) Optical microscopy images ofα-phase crystals on quartz substrate annealed at 160 °C (left) and 180 °C (right). Scale bar, 100 μm. (b) XRD patterns of theα-phase crystals on a quartz substrate as a function of annealing temperature between 25 °C and 230 °C. (c) DSC ofα-phase with different heating rates of 10 °C min−1(blue), 2 °C min−1(red) and 1 °C min−1(black), respectively. The weight of samples is about 2 mg. (d) Ultraviolet–visible absorption spectra of 10−5mol l−1chloroform solution (black) andα- andβ-phase crystals.α-phase crystals were grown from solution and washed by methanol, then dropped on quartz substrate (blue).β-phase crystals were prepared on quartz substrate by sublimation under ambient conditions (magenta). Inset: structural transition inside the molecular layer. Figure 3: Observations upon phase transformation from α -phase to β -phase. ( a ) Optical microscopy images of α -phase crystals on quartz substrate annealed at 160 °C (left) and 180 °C (right). Scale bar, 100 μm. ( b ) XRD patterns of the α -phase crystals on a quartz substrate as a function of annealing temperature between 25 °C and 230 °C. ( c ) DSC of α -phase with different heating rates of 10 °C min −1 (blue), 2 °C min −1 (red) and 1 °C min −1 (black), respectively. The weight of samples is about 2 mg. ( d ) Ultraviolet–visible absorption spectra of 10 −5 mol l −1 chloroform solution (black) and α - and β -phase crystals. α -phase crystals were grown from solution and washed by methanol, then dropped on quartz substrate (blue). β -phase crystals were prepared on quartz substrate by sublimation under ambient conditions (magenta). Inset: structural transition inside the molecular layer. Full size image The structural phase transformation was further investigated by DSC, which confirmed the solid-to-solid transition at a temperature around 180 °C ( Fig. 3c ). Notably, no second endothermic peak could be observed in the heating process, because the crystals do not melt but sublime at higher temperature. The facts that also no exothermic transition is observed upon cooling and that neither endothermic nor exothermic transitions are observed in subsequent thermal cycles ( Supplementary Fig. 8 ) suggest that complete transition from α -phase to β -phase occurs during the first thermal cycle and that the β -phase does not transform into α -phase during the time scale and in the temperature range of this experiment. This combined POM, DSC and XRD studies indicate that at temperatures >160 °C the original α -phase crystals are in a metastable state and that the β -phase crystals are the thermodynamically favoured polymorph at elevated temperature ( Fig. 3b ). Upon further increase of temperature, the (h00) peaks of α -phase disappeared completely despite of the fact that the ribbon-shaped crystals appeared still to co-exist on the quartz substrate. A closer view on the ribbon-shaped crystals’ surface revealed that the original ribbon-shaped crystals are indeed destroyed and are now composed of many small grains of β -phase crystals ( Supplementary Fig. 6i ). The transformation of the α -phase crystals at elevated temperatures can be well explained by the decrease in entropy [27] , as the unit cell of the α -phase, which contains two identical NDI molecules, is converted to a unit cell of the β -phase containing only one NDI isomer. In addition, extrapolating the thermal expansion deduced from the crystal structure at 100 and 200 K ( Supplementary Table 1 ) the β -polymorph is expected to be the lower density phase at the transition temperature of about 165 °C with a cell volume of about 615.5 Å 3 (per one molecule) compared with the α -phase with 1,212.6 Å 3 (per two molecules). Accordingly, the β -phase allows for lattice vibrations of larger amplitudes and a higher occupation density. By the result above, the transformation from α -phase to β -phase can be easily realized by heating ( Fig. 3 and Supplementary Fig. 6 ). Inspired by the fact that β -phase crystals were not stable at low temperature and only showed very weak diffraction patterns when collecting the single-crystal structural data at low temperatures, the reverse pathway of realizing transition from β - to α -phase has been successfully demonstrated by keeping the yellow coloured β -phase crystals in a closed vial in liquid nitrogen for several months ( Supplementary Figs 9 and 10 ). The more complex diffraction patterns indicated that the phase transformation from β - to α -phase crystals occurred only partially, resulting in a polymorphous sample. Unfortunately, single-crystal XRD spots from β - to α -phase could not be detected at the temperature of 100 K even after hours. Maybe harsher conditions, for example, high pressure, are needed for the fast and fully thermal-induced transformation of large crystals from β - to α -phase. During our crystal growth experiments, we were stunned by the fact that solution-grown α -phase crystals appeared colourless, whereas sublimation-grown β -phase crystals appeared yellowish. Accordingly, we investigated the ultraviolet–visible absorption properties of both polymorphs and compared the results with Cl 2 -NDI in CHCl 3 solution ( Fig. 3d ). At the chosen low concentration of 10 −5 mol l −1 , Cl 2 -NDI molecules are present as monomers in CHCl 3 , which show absorption peaks at 358, 382 and 403 nm. Very similar absorption bands are observed for the α -phase crystal whose longest wavelength transition is only blue-shifted by 2 nm. In contrast, the β -phase crystals show a pronounced red-shift of 10 nm and the 413 nm peak is clearly the one of highest intensity. These spectral shifts can indeed be well rationalized by excitonic coupling of Cl 2 -NDI molecules in the unit cell of the respective polymorph [38] . Thus, the closest neighbour Cl 2 -NDI molecules are stacked with a slipping angle of 62° and 41° for α - and β -phase, respectively. For a slipping angle larger than 54.7° (magic angle) a blue shift is expected (H-type coupling), whereas for a slipping angle smaller than 54.7° a red-shift is expected (J-type coupling) [39] . In the present case, the spectral shifts are, however, only modest because the transition dipole moments of these NDIs are rather small and the slipping angles are close to the magic angle ( Supplementary Fig. 11a ). Also the polarization-induced red-shift upon crystal formation [40] obviously over-compensates the blue-shift for the α -phase, leading to almost identical spectra in the crystal and in solution. As expected from previous studies, we could also follow the transformation from α - to β -phase by temperature-dependent ultraviolet–visible spectroscopy ( Supplementary Fig. 11b ). Single-crystal and thin-film field-effect transistors Although both polymorphs exhibit the same Cl 2 -NDI chemical structure, the differences in molecular packing and in particular in π–π orbital overlap suggest different charge transport properties for these two single crystals. The single-crystal transistors on Si/SiO 2 substrate were fabricated by sublimation in air and electrode contacting by adhesive gold film method ( Fig. 4a ) [41] . Like for the previously reported α -phase single crystals [35] , devices based on β -phase single crystals exhibited air-stable n-type transistor behaviour in combination with Au contacts. The average performances obtained from 22 devices on Si/SiO 2 yield a mobility of 2 cm 2 V −1 s −1 , a threshold voltage of 8 V and an on/off current ratio of 10 6 ( Supplementary Table 2 ). For the best device on Si/SiO 2 substrate whose transfer curve is depicted in Fig. 4b (for output curves, see Supplementary Fig. 12 and AFM cross-section analysis Supplementary Fig. 13 ), the mobility is 3.25 cm 2 V −1 s −1 , the threshold voltage 7 V and the on/off current ratio 8 × 10 6 . The versatility of such simple sublimation of an organic semiconductor molecule in air without expensive vacuum instrumentation was further demonstrated by the evaporation of Cl 2 -NDI at a temperature of 280 °C and deposition on a 2 mm distant SiO 2 wafer, yielding highly crystalline thin films with large domain sizes. OTFTs prepared from these films through deposition of gold contacts through a shadow mask afforded bottom-gate, top-contact configuration OTFTs with excellent average mobility of 0.37 cm 2 V −1 s −1 , threshold voltage of 3 V and on/off current ratio >10 5 under ambient conditions (see Supplementary Fig. 14 ). 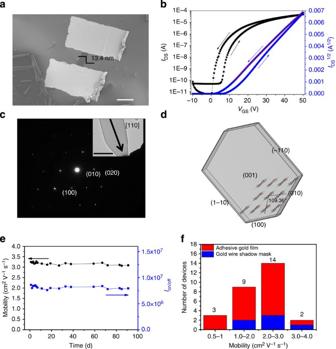Figure 4:β-phase single-crystal field-effect transistors. (a) Scanning electron microscopy image ofβ-phase single-crystal transistor fabricated by adhesive gold film method on Si/SiO2, and theW/Lof channels is 25.51/59.91 μm. Scale bar, 50 μm. (b) Corresponding transfer curve. (c) SAED patterns ofβ-phase single crystal (inset: transmission electron microscopy image. Scale bar, 2 μm.). (d) Bravais-Friedel-Donnay-Harker (BFDH) crystal morphology ofβ-phase. The energetically preferred growth of the crystal is along the [110] direction. For clarity, fluoroalkyl chains were omitted. (e) The stability of one representative device stored and measured in air at room temperature (mobility in black, on/off ratio in blue). (f) Mobility distribution of 28 SCFETs (22 on Si/SiO2substrate by adhesive gold film method in red and 6 on OTES-modified substrate by gold wire shadow mask method in blue). Figure 4: β -phase single-crystal field-effect transistors. ( a ) Scanning electron microscopy image of β -phase single-crystal transistor fabricated by adhesive gold film method on Si/SiO 2 , and the W / L of channels is 25.51/59.91 μm. Scale bar, 50 μm. ( b ) Corresponding transfer curve. ( c ) SAED patterns of β -phase single crystal (inset: transmission electron microscopy image. Scale bar, 2 μm.). ( d ) Bravais-Friedel-Donnay-Harker (BFDH) crystal morphology of β -phase. The energetically preferred growth of the crystal is along the [110] direction. For clarity, fluoroalkyl chains were omitted. ( e ) The stability of one representative device stored and measured in air at room temperature (mobility in black, on/off ratio in blue). ( f ) Mobility distribution of 28 SCFETs (22 on Si/SiO 2 substrate by adhesive gold film method in red and 6 on OTES-modified substrate by gold wire shadow mask method in blue). Full size image In order to better compare with previously studied α -phase single-crystal transistors on OTES substrate [35] , the same device architecture was used for β -phase crystals grown on OTES-modified substrate by gold wire mask method. For six devices, a quite similar mobility distribution is obtained as for the previous 22 devices ( Fig. 4f ) and also the characteristic transistor data of the best device are pretty similar: mobility of 3.5 cm 2 V −1 s −1 , threshold voltage of 7 V and the on/off ratio of 10 8 ( Supplementary Table 2 and Supplementary Fig. 15 ). Although these mobility values are quite impressive, they are about a factor of two lower than those reported in our previous work on α -phase single-crystal transistors (highest mobility of 8.6 cm 2 V −1 s −1 , threshold voltage of 9 V and on/off ratio of 7 × 10 7 ) [35] . To make sure that the measured direction of transport complies with the same alignment of molecular packing related to the direction of crystal growth, we performed selected-area electron diffraction (SAED) studies that showed that the fastest growth direction for the β -phase crystals occurs along the [110] direction, which is the same as in case of α -phase—the orientation of π-stacking ( Fig. 4c and d ). Although the α -phase crystals showed the higher mobility, a notable advantage given by β -phase crystals is their outstanding ambient stability. Thus, keeping the device in air over 3 months, less degradation of β -phase devices (5%, Fig. 4e ) is observed compared with α -phase SCFETs (13%) [35] . With these results we can conclude that SCFETs for both α -phase and β -phase single crystals exhibit excellent electron transport capabilities along the direction of fastest crystal growth. As shown in Fig. 4 and ref. 34 , respectively, this direction complies with the [110] direction for the β -phase and the [001] direction of π-stacking for the α -phase. By its two-dimensional brick-wall packing and the resulting slipping angles of 41° and 32°, the β -phase exhibits a weaker electronic coupling between the π-scaffolds of neighbouring molecules and a longer percolation pathway for electrons to cross the unit cell compared with the α -phase with its more directional coupling and transport along the π-stacks. Therefore, the higher mobility observed for the α -phase can be rationalized by the deviation between the investigated current direction and the direction of highest mobility in the β -phase crystals. This conclusion is supported by the slower degradation rate of the β -phase SCFETs assuming an identical degradation rate per molecule for both polymorphs. In case of a rather one-dimensional transport ( α -phase), any structural or chemical defect limits the overall current, whereas for a more two-dimensional transport ( β -phase), an alternative percolation path can bypass such defects. Temperature-dependent transistor performances of two phases It is well known that the thermal-induced defects in crystals have a great influence on device performance, reflecting in mobility and threshold voltage [42] , [43] , [44] . This issue might be particularly relevant in situations like here where temperature-dependent structural phase transitions may be present. Accordingly, device performances were characterized from room temperature to 90 °C that basically satisfies temperature changes by heat produced during operation in practical application ( Fig. 5 ). For the α -phase SCFETs, a reduction in source-drain current occurred leading to a drop of mobility from 5.2 cm 2 V −1 s −1 at 40 °C to 1.6 cm 2 V −1 s −1 at 90 °C and this decrease is irreversible when cooling down to room temperature ( Supplementary Table 3 ). In contrast, β -phase SCFETs showed excellent air-stability in the whole temperature range up to 90 °C. Indeed, the source-drain currents even showed some slight increase and the turn-on voltage some slight decrease with increasing temperature, leading to the highest mobility of 3.1 cm 2 V −1 s −1 at a temperature of 65 °C and the lowest threshold voltage of 1 V at a temperature of 90 °C ( Supplementary Table 3 ). A possible rationale for these observations is provided by the competition between thermal-induced trap states, for example, by lattice distortions [42] , [43] and an enhanced thermal-activated hopping transport [44] . At the temperature of 90 °C, α -phase crystals can be regarded as metastable phase as they show a release of elastic energy upon volume expansion. Therefore, more charge traps associated with crystal defects originate by the onset of the thermal-induced transformation of α -phase to β -phase crystals, especially between the (h00) molecular planes. Owing to the lattice distortions, a greater influence on charge injection can be observed for α -phase than for β -phase SCFETs. Furthermore, higher mobility and lower threshold voltage for β -phase SCFETs are supported by the lower thickness of these crystals, resulting in higher injection field strengths at similar gate voltage and shorter charge carrier pathways towards the accumulation layers being relevant for electron transport. 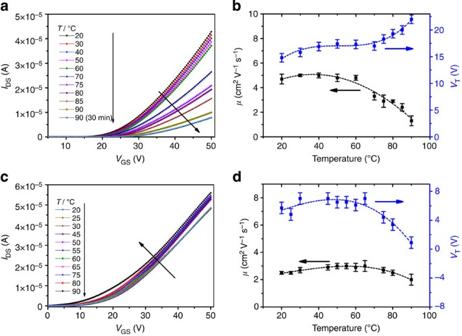Figure 5: Temperature-dependent SCFET performance. Drain current as a function of temperature with a heating rate of about 2 °C min−1for representativeα-phase (a) and forβ-phase (c) SCFETs. (b) Corresponding mobility (black) and threshold voltage (blue) changes with temperature for representativeα-phase (b) and forβ-phase (d) SCFETs. Error bars inb,drepresent standard deviation from the linear regression analysis of (IDS(VGS))1/2atVDS=50 V and the dotted lines are a guide to the eye. Figure 5: Temperature-dependent SCFET performance. Drain current as a function of temperature with a heating rate of about 2 °C min −1 for representative α -phase ( a ) and for β -phase ( c ) SCFETs. ( b ) Corresponding mobility (black) and threshold voltage (blue) changes with temperature for representative α -phase ( b ) and for β -phase ( d ) SCFETs. Error bars in b , d represent standard deviation from the linear regression analysis of ( I DS ( V GS )) 1/2 at V DS =50 V and the dotted lines are a guide to the eye. Full size image This is the first report on the growth of n-channel organic thin film and organic single-crystal transistors by sublimation at ambient pressure in air. Such sublimation under ambient condition offers a very simple and inexpensive processing procedure that should be also applicable to other small organic semiconductor molecules that exhibit good chemical and thermal robustness combined with a low molecular weight as required for sublimation at reasonable temperatures. Most remarkably, in combination with contacts attached by the technique of adhesive gold film, not even vacuum equipment is needed for the whole process from the crystals growth, device fabrication and transistor operation of Cl 2 -NDI SCFETs. In contrast to inkjet printing [6] , no organic solvent, no additives to meet rheological demands for high-quality printing as well as post annealing treatments of the active layer are required for the processing of small organic semiconductors by evaporation in air. Therefore, we hope that our new approach will open up new opportunities in sublimation-assisted dye processing on technological scales and thus bring great prospect in the field of organic electronics. In addition, we discovered that these single crystals grown by sublimation constitute a new polymorph of the record ambient n-channel charge carrier material Cl 2 -NDI. In contrast to the herringbone packing reported before, the new phase of Cl 2 -NDI exhibits two-dimensional brick-wall packing mode. Based on temperature-dependent XRD, DSC, ultraviolet–visible studies and supported by SAED and X-ray characterization of single crystals, the two polymorphs could be assigned as α -phase and β -phase. Both phases exhibit excellent transistor performance in SCFETs on OTES-modified substrate at room temperature under ambient conditions with electron mobilities of up to 8.6 cm 2 V −1 s −1 for α -phase and up to 3.5 cm 2 V −1 s −1 for β -phase. However, although the performance of the α -phase SCFETs decreased upon increasing temperature, the β -phase SCFETs showed excellent stability even at 90 °C in air. Furthermore, β -phase SCFETs and OTFTs exhibit high performance on simple Si/SiO 2 substrates with mobilities up to 3.25 cm 2 V −1 s −1 and 0.37 cm 2 V −1 s −1 , respectively. By establishing a correlation between crystal structures and their device performance, we further obtained insight into percolation pathways and packing structure-transport property relationships. Growth of single crystals and SCFET fabrication The synthesis of Cl 2 -NDI and the growth of α -phase crystals had been described in the earlier literature [31] , [35] . The β -phase single crystals were grown by sublimation at ambient pressure in air and then deposited on Si/SiO 2 substrate. The detailed steps are as follows: a droplet (60 μl) of Cl 2 -NDI in chloroform with the concentration of 1 mg ml −1 was dropped onto Si/SiO 2 and the solvent was allowed to evaporate to give a thin film with a thickness of tens of micrometres. Then, the Si/SiO 2 substrate covered with Cl 2 -NDI thin film was put on a heating stage at a temperature of 180 °C for 20 min. The molecules sublimed and deposited as crystalline ribbons on the surface of the opposing substrate (Si/SiO 2 or OTES-modified Si/SiO 2 ). The surface density and thickness of the crystals were controlled by adjusting the distance between the bottom Si/SiO 2 with the Cl 2 -NDI thin film and the top substrate for crystal growth. In our experiment, the distance between the substrate with a drop-casted Cl 2 -NDI thin film on top of the heating stage and the substrate was about 5.7 mm to achieve a temperature difference of 30±1 °C between heating stage and substrate. Most crystals with a thickness of below 50 nm were obtained after 20 min deposition at 180 °C. A heavily doped Si wafer with a SiO 2 layer of 100 nm with and without OTES self-assembled monolayer ( C i =34 nF cm −2 ) served as the bottom-gate electrode and dielectric layer for the SCFET fabrication, respectively. Electrode contacts were either manufactured by adhesive gold flakes or gold wire shadow mask methods, respectively, to give bottom-gate top contact single-crystal field-effect transistors [35] . Organic thin-film transistor fabrication A few milligrams of Cl 2 -NDI were deposited in a molybdenum crucible. The crucible was put on a hot plate mounted on an automated, mechanical stage, which allows a controlled, lateral movement at a constant velocity in the range of 0.5–16 mm s −1 . When the hot plate was heated to 280 °C, the material started to evaporate as became visible by rising vapour. Next, a silicon wafer, covered with a 300 nm thick layer of silicon dioxide ( C i =11 nF cm −2 ) was heated on a second hot plate to 170 °C. Meanwhile, the hotplate supporting the crucible was started to move with a constant speed of 10 mm s −1 . The preheated substrate was then removed from the hotplate and immediately held top-down in the vapour of the moving crucible. The distance between the substrate and the moving crucible was 2 mm. After moving through the vapour, a polycrystalline layer of the compound could be found on the surface of the silicon dioxide. The deposited layer was highly crystalline with domain-sizes of 5–20 μm. The thickness of the polycrystalline layer was measured by a profilometer to be around 50 nm. Next, the source and drain contacts were patterned on the organic layer, by vacuum-evaporation of a 50-nm-thick layer of gold through a shadow mask. The resulting transistors had a channel length ( L ) of 100 μm and a channel width ( W ) of 200 μm. Device characterization The current–voltage characteristics of the SCFETs were recorded using an Agilent 4155C semiconductor parametric analyzer (Agilent Technologies, Inc.) with heating stage system under ambient condition. All transfer curves were measured either at V DS =50 V and V GS =0–50 V (SCFETs) or at V DS =40 V and V GS =−20–60 V (OTFTs). The carrier mobilities of the SCFETs were calculated in the saturation regime from the plot of the square root of the source-drain current ( I DS ) versus the gate-source voltage ( V GS ) by fitting the data to the equation μ =(2 I DS L /[ WC i ( V GS - V T ) 2 ]), where L and W represent channel length and the width of the crystal, respectively. C i is the capacitance per unit area of the dielectric insulator and V T is the threshold voltage. Atomic force microscopy The thickness and surface morphology of crystals were measured by AFM at ambient conditions with a NT-MDT Solver Next system in semi-contact mode. Ultraviolet–visible absorption spectroscopy Ultraviolet–visible spectra were acquired on a Lambda 950 instrument (Perkin-Elmer) with an Ulbricht sphere. The temperature-dependent ultraviolet–visible spectra were carried out by Maya2000 Pro diode array spectrometer (Ocean Optics) with reflection probe and Gestigkeit PZ28-2 precision heating stage. Differential scanning calorimetry DSC measurements were carried out by TA instruments Q1000. Polarization optical microscopy POM images were taken by Olympus BX41 with heating system. X-ray spectroscopy Single-crystal X-ray data were collected on a Bruker D8Quest Kappa Diffractometer using CuKα radiation from an Incoatec IμS microsource with Montel multi-layered mirror, a Photon100 CMOS detector and Apex2* software. Temperature-dependent wide-angle X-ray scattering experiments were carried out using a Bruker Nanostar Diffractometer using CuKα radiation ( λ =1.5418 Å). Powder X-ray diffraction studies were carried out with a Bruker D8 diffractometer using CuKα radiation ( λ =1.5418 Å). The data were collected using a Ni-filtered Cu-target tube at room temperature in the 2 θ range from 3° to 30°. Scanning electron microscopy Scanning electron microscopy images were recorded using a Ultra plus field emission scanning electron microscope (Carl Zeiss) equipped with GEMINI e-beam column operated at 5 kV. Transmission electron microscopy Transmission electron microscopy and SAED measurements were carried out on a JEOL 2010 with an accelerating voltage of 100 kV. Cl 2 -NDI microcrystals were prepared on a carbon-covered copper grid by sublimation at ambient pressure in air. How to cite this article: He, T. et al . Single-crystal field-effect transistors of new Cl 2 -NDI polymorph processed by sublimation in the air. Nat. Commun. 6:5954 doi: 10.1038/ncomms6954 (2015). Accession codes: The X-ray crystallographic coordinates for structures reported in this article have been deposited at the Cambridge Crystallographic Data Centre (CCDC), under deposition number CCDC 1018034 to 1018036. These data can be obtained free of charge from the CCDC via www.ccdc.cam.ac.uk/data_request/cif .